A female gametocyte-specific ABC transporter plays a role in lipid metabolism in the malaria parasite ATP-binding cassette (ABC) transporters serve a variety of physiological functions as well as play key roles in drug resistance. The genome of the human malaria parasite, Plasmodium falciparum , encodes multiple members of this family, one of which, gABCG2, is transcribed predominantly in the gametocyte stage. Here we use gene deletion and tagging to investigate the expression, localization and function of gABCG2. The protein is found in a single dot-like lipid-rich structure within female, but not male, gametocytes. gABCG2-knockout cell lines produce more gametocytes of both sexes. By contrast, cholesteryl esters, diacylglycerols and triacylglycerols are significantly reduced in gABCG2-knockout gametocyte stages. We propose a role for gABCG2 in the regulation of gametocyte numbers and in the accumulation of neutral lipids, which are likely important for parasite development in the insect stages of the parasite life cycle. Malaria is an infectious disease, caused by parasites of the genus Plasmodium and transmitted by the female Anopheles mosquito. P. falciparum is the most virulent of the five species of malaria parasite known to infect humans and it accounts for the vast majority of the estimated 627,000 annual deaths from malaria ( http://www.who.int/malaria/publications/world_malaria_report_2013/en/ ). In the course of its complex life cycle, the parasite invades the erythrocytes of its mammalian host. The majority of the intraerythrocytic parasites are asexual. However, a small proportion differentiate into sexual, male or female, forms known as gametocytes. It is through the ingestion of gametocytes, in the course of the mosquito vector taking a blood meal, that the parasite is transmitted from its vertebrate to its invertebrate host. The differentiation of a small proportion of the asexual blood-stage parasites into the transmissible sexual form (‘gametocytogenesis’) is a crucial ‘bottleneck’ step in the parasite life cycle, and in the transmission of the disease from one person to another [1] . However, the molecular mechanisms involved are largely unknown [2] and progress in the field has been hindered by the combination of the paucity of suitable gametocyte-specific marker molecules, and the fact that only a small subset of asexual forms undergo differentiation to the sexual forms. Differentiation involves an initial ‘commitment’ step, after which the parasites develop through five distinctive gametocyte stages (I–V) into transmissible male and female gametes over a period of 10–14 days [3] . The male/female ratio in the P. falciparum gametocyte population tends to be female biased, with both strain-specific and environmental factors playing a role in determining the actual ratio [2] . A number of antimalarial drugs (including chloroquine and sulphadoxine-pyrimethamine), while killing the asexual forms of the parasite, induce gametocyte formation and may result in increased transmission potential [3] . None of the ‘sex-specific’ markers characterized to date is genuinely ‘specific’; they are not expressed exclusively in males or females. Rather, they show different levels of expression in the two different gametocyte forms. The ATP-binding cassette (ABC) proteins constitute a large family of transmembrane proteins that transport a diverse range of substrates including amino acids, lipids, inorganic ions, proteins and sugars [4] . ABC transporters play a key role in multidrug resistance (MDR), both in human cancer cells and in pathogenic microbes [5] , [6] . The P. falciparum genome encodes 11 putative ABC transporter proteins [7] . Thus far, Plasmodium ABC proteins have been studied in the context of their prominent roles in conferring drug resistance. One of these ABC proteins, the P. falciparum MDR protein 1, was reported to be linked to chloroquine resistance [8] and later shown to modulate susceptibility of cultured P. falciparum parasites to multiple compounds [6] . Alleles encoding two additional ABC transporters, the MDR-associated protein and the MDR protein 2, were associated with altered resistance to 4-aminoquinolines, for example, quinine and chloroquine, and toxic metal ions, respectively [9] , [10] . However, the physiological role(s) of these ABC transporters remains unknown. An analysis of the expression profiles of the ABC proteins encoded by P. falciparum (throughout the intraerythrocytic cycle) has revealed that for one of these (PlasmoDB accession number PF3D7_1426500, referred to here as gABCG2), expression of the encoding RNA is largely restricted to the gametocyte stage ( http://www.plasmodb.org/ ) [11] . Here we explore the expression, localization and function of gABCG2 in all stages of the parasite’s erythrocytic phase of the life cycle. The results are consistent with this transporter playing a role both in lipid metabolism and in the process of parasite commitment to gametocytogenesis. gABCG2 is expressed in gametocytes and early ring-stage parasites BLAST searches identified gABCG2, encoded by the PF14_0244 gene, as a member of the G-subgroup of the ABC family (ABCG) with orthologues in other Plasmodium species (PlasmoDB accession number PF3D7_1426500). The orthologues in the species infecting humans ( P. falciparum , P. knowlesi , P. vivax ) form a separate branch to those in the rodent malaria species ( Supplementary Fig. 1 ). The closest group outside of the genus Plasmodium are genes encoding ABCG transporters in plants. To monitor expression of the gABCG2 protein, we used a 3′ replacement strategy to generate 3D7 parasites expressing gABCG2 protein fused to a green fluorescent protein (GFP). Expression of this chimeric protein was under the control of the endogenous gABCG2 promoter ( Supplementary Fig. 2A ). Western blot analysis using an anti-GFP antibody revealed that the chimeric protein was expressed at detectable levels in gametocytes as early as stage II (4 days post-commitment) and could be detected in all subsequent gametocyte stages, as well as in gametes ( Fig. 1a ). Western blot analyses of asexual (ring, trophozoite and schizont) parasite populations failed to detect the protein. However, quantitative reverse transcription PCR analysis of the different stages of wild-type parasites revealed the presence of gABCG2 transcripts in ring-stage parasites ( Fig. 1b ), albeit at a lower level than was seen in gametocyte populations. 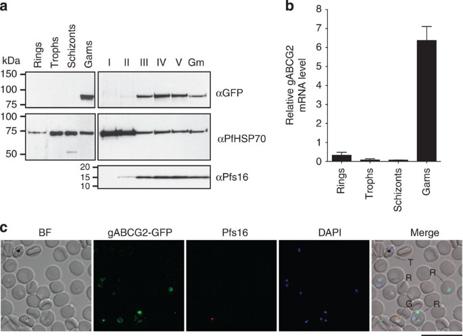Figure 1: gABCG2 is expressed in early rings and gametocytes. (a) Western blot performed on the synchronous GFP-tagged parasite (pGREP-1/PfgABCG2) samples of different life cycle stages using anti-GFP antibody. The membranes were also probed with anti-PfHSP70 antibody as a loading control. Antibody against Pfs16 was used as a marker of gametocytes. I–V, gametocytes stage 1 to stage 5. Gm, gametes. For full-sized western blots, seeSupplementary Fig. 7. (b) Relative expression of gABCG2. Quantitative real-time PCR was performed using a probe and primer set specific for gABCG2 on synchronous wild-type parasite samples. PFL2215w (ActinI) was used as a reference gene since the amount of mRNA for this gene is constant across all parasite stages62. Values are mean (±s.d.) of triplicate independent samples. (c) Immunofluorescence microscopy of paraformaldehyde/glutaraldehyde-fixed GFP-tagged gABCG2 parasites probed with anti-GFP (green) and anti-Pfs16 (red) antisera. The nuclei were visualized with DAPI. R, ring; T, trophozoite; G, gametocyte. Scale bar, 25 μm. Figure 1: gABCG2 is expressed in early rings and gametocytes. ( a ) Western blot performed on the synchronous GFP-tagged parasite (pGREP-1/PfgABCG2) samples of different life cycle stages using anti-GFP antibody. The membranes were also probed with anti-PfHSP70 antibody as a loading control. Antibody against Pfs16 was used as a marker of gametocytes. I–V, gametocytes stage 1 to stage 5. Gm, gametes. For full-sized western blots, see Supplementary Fig. 7 . ( b ) Relative expression of gABCG2. Quantitative real-time PCR was performed using a probe and primer set specific for gABCG2 on synchronous wild-type parasite samples. PFL2215w (ActinI) was used as a reference gene since the amount of mRNA for this gene is constant across all parasite stages [62] . Values are mean (±s.d.) of triplicate independent samples. ( c ) Immunofluorescence microscopy of paraformaldehyde/glutaraldehyde-fixed GFP-tagged gABCG2 parasites probed with anti-GFP (green) and anti-Pfs16 (red) antisera. The nuclei were visualized with DAPI. R, ring; T, trophozoite; G, gametocyte. Scale bar, 25 μm. Full size image When viewed under the microscope, a specific GFP signal could be detected in early ring stages; this was lost on maturation of the parasite into the late ring stage. To distinguish between rings that produce asexual forms and rings destined to become gametocytes, we co-stained populations in immunofluorescence assays with antibodies against GFP and Pfs16, one of the earliest known markers of gametocyte commitment [12] . A GFP signal was observed both in early rings that did not co-stain with Pfs16 and those that co-stained with Pfs16 (and were therefore destined for development into gametocytes; Fig. 1c ). Expression of gABCG2 in rings is therefore not a marker for subsequent gametocyte development. Due to the small size of the young ring parasites, it was difficult to determine the exact localization of the GFP signal; however, the gABCG2-GFP-fusion protein appeared to accumulate in several punctae in the cytoplasm of the ring-stage parasite. These results indicate low-level expression of gABCG2 in very early ring stages and higher-level expression in gametocytes. Female-specific expression and location in a single punctate structure Parasites expressing gABCG2-GFP were induced to form gametocytes by growing cultures to high parasitemia, then enriching the cultures by N-acetyl- D -glucosamine (GluNAc) treatment and magnet purification. GFP fluorescence was observed from stage I gametocytes onwards in distinct small round structures of ~0.5 μm diameter ( Fig. 2a ). 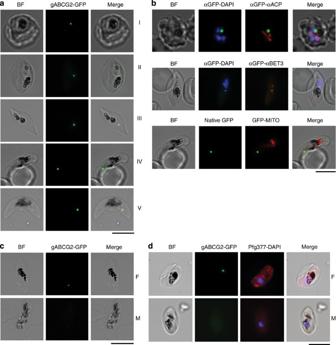Figure 2: gABCG2 is observed as a single spot close to the DV in female gametocytes. (a) Live-cell fluorescence microscopy of GFP-tagged gABCG2 gametocytes was performed for the five gametocyte development stages (I–V). (b) Immunofluorescence microscopy of paraformaldehyde/glutaraldehyde-fixed GFP-tagged gABCG2 parasites probed with anti-GFP (green) and anti-ACP (apicoplast marker), anti-BET3 (Golgi marker) antisera and MitoTracker (red). (c) Live-cell fluorescence microscopy of a GFP-tagged gABCG2 transfectant. Mature male and female gametocytes were differentiated on the basis of the different patterns of hemozoin distribution. (d) Immunofluorescence microscopy of paraformaldehyde/glutaraldehyde-fixed GFP-tagged gABCG2 parasites probed with anti-GFP (green) and anti-Pfg377 (red) antisera. The nuclei were visualized with DAPI (violet). The data are typical of those obtained from at least 100 cells. BF, bright field. Scale bar, 5 μm. Figure 2: gABCG2 is observed as a single spot close to the DV in female gametocytes. ( a ) Live-cell fluorescence microscopy of GFP-tagged gABCG2 gametocytes was performed for the five gametocyte development stages (I–V). ( b ) Immunofluorescence microscopy of paraformaldehyde/glutaraldehyde-fixed GFP-tagged gABCG2 parasites probed with anti-GFP (green) and anti-ACP (apicoplast marker), anti-BET3 (Golgi marker) antisera and MitoTracker (red). ( c ) Live-cell fluorescence microscopy of a GFP-tagged gABCG2 transfectant. Mature male and female gametocytes were differentiated on the basis of the different patterns of hemozoin distribution. ( d ) Immunofluorescence microscopy of paraformaldehyde/glutaraldehyde-fixed GFP-tagged gABCG2 parasites probed with anti-GFP (green) and anti-Pfg377 (red) antisera. The nuclei were visualized with DAPI (violet). The data are typical of those obtained from at least 100 cells. BF, bright field. Scale bar, 5 μm. Full size image In an attempt to localize the GFP signal, the gABCG2-GFP-expressing parasites were screened with markers of known Plasmodium organelles ( Fig. 2b ). The signal for the labelled structure did not co-localize with antibodies against acyl-carrier protein (ACP; an apicoplast marker [13] ), antibodies against the ‘blocked early in transport’ protein (BET3; a Golgi apparatus marker [14] ) or MitoTracker (a marker for mitochondria). Hence, gABCG2 is not associated with these organelles. The fluorescence was restricted to female gametocytes; there was no GFP fluorescence observed in male gametocytes ( Fig. 2c ). Female gametocytes were identified by the more tightly compartmentalized localization of hemozoin ( Fig. 2c ) [15] as well as the increased presence of Pfg377, a marker of osmiophilic bodies of which there are more in female than in male gametocytes [16] ( Fig. 2d ). The majority of female gametocytes had a single fluorescent structure. On very rare occasions, there were two of these structures per cell. In stage I and stage II female gametocytes, the fluorescent structure was observed to be located near the digestive vacuole (DV). From stage III onwards, the structure was disconnected from the DV and had moved towards the apical end of the gametocyte. In mature (stage IV) gametocytes, the structure had increased in size, to ~1 μm diameter. The gABCG2-associated structure is rich in neutral lipids ABC proteins commonly transport lipophilic solutes, including lipids themselves [17] . To see whether the gABCG2 transporter co-localizes with any lipid-containing structures, we stained gABCG2-GFP-expressing gametocytes with Nile red, a lipophilic stain [18] . Nile red stains neutral lipid-containing structures within the cytoplasm of asexual parasites, highlighting in particular small cytoplasmic lipid droplets located adjacent to the exterior of the DV [19] . What becomes of these structures during the development of gametocytes is unknown. In gametocytes, the GFP signal of the gABCG2-GFP co-locates with a large Nile red-stained structure near the DV ( Fig. 3a ). This structure is ~1 μm in diameter, with gABCG2 localized to its periphery. The same structure was detected when gABCG2-GFP parasites were stained with another neutral lipid stain (HCS Lipid TOX Red neutral lipid stain) and with Bodipy-TR-ceramide, which is commonly used as a lipid marker [20] . Super-resolution microscopy performed on Bodipy-TR-ceramide-stained gABCG2-GFP-expressing parasites revealed a more heterogenous distribution of the gABCG2 within the round structure ( Fig. 3b ; Supplementary Movie 1 ). The heterogenous distribution of gABCG2-GFP was observed in all of the <50 analysed female gametocytes and could be detected in stage III, IV and V gametocytes in both fixed- and live-cell preparations ( Supplementary Fig. 3 ). 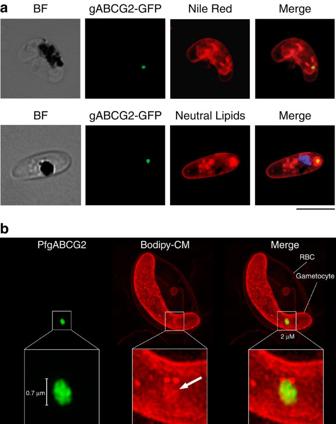Figure 3: Association of gABCG2 with lipids. (a) Fluorescence microscopy of formaldehyde-fixed GFP-tagged gABCG2 gametocytes labelled with Nile red (top) or neutral lipid (bottom) stains. The nuclei were visualized with DAPI (blue). (b) 3D-SIM of a representative BODIPY-TR-ceramide-labeled gametocyte. A maximum intensity projection of a stack is displayed. The arrow indicates a lipid-rich structure. RBC, red blood cell membrane. Figure 3: Association of gABCG2 with lipids. ( a ) Fluorescence microscopy of formaldehyde-fixed GFP-tagged gABCG2 gametocytes labelled with Nile red (top) or neutral lipid (bottom) stains. The nuclei were visualized with DAPI (blue). ( b ) 3D-SIM of a representative BODIPY-TR-ceramide-labeled gametocyte. A maximum intensity projection of a stack is displayed. The arrow indicates a lipid-rich structure. RBC, red blood cell membrane. Full size image Disruption of gABCG2 results in a reduction in neutral lipids To assess the function of gABCG2 in P. falciparum , we generated parasites in which the corresponding gene locus (PF14_0244) was disrupted by transfecting the pCC-1/ PfgABCG2 plasmid into P. falciparum 3D7-infected erythrocytes, leading to homologous recombination and double-crossover recombination (see Supplementary Fig. 4A for schematic strategy) [21] . Southern blot analysis revealed an absence of wild-type bands in the transfected, drug-selected cell lines, with new DNA fragment sizes of around 3.7 kb for the 5′ flank and 3.6 kb for the 3′ flank, indicating the correct integration of the resistance cassette and consequent disruption of the PF14_0244 locus ( Supplementary Fig. 4B ). The knockout (ΔgABCG2) parasites were subjected to a lipidomic analysis using nanoelectrospray ionization (ESI) tandem mass spectrometry (MS), to assess whether the absence of gABCG2 (ΔgABCG2) had any effect on the lipid composition of the parasitized erythrocytes. A comparison of lipid profiles of erythrocytes infected with asexual (trophozoite-stage) parasites revealed no significant differences between wild-type and ΔgABCG2 parasites ( Fig. 4a ). This analysis also revealed that the amphipathic lipids that typically constitute eukaryotic membranes, that is, free cholesterol (FC), phosphatidylcholine (PC) and phosphatidylethanolamine (PE), are present in trophozoite-infected erythrocytes with PC being the major (~30%) component. 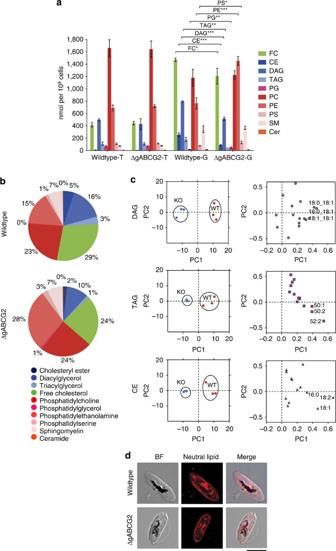Figure 4: Altered lipid composition in gABCG2-knockout parasites. (a) Lipid profile of gABCG2-disrupted trophozoite (ΔgABCG2-T) and stage IV gametocyte (ΔgABCG2-G) compared with wild type. T, trophozoite; G, gametocyte; PG, phosphatidylglycerol; PS, phosphatidylserine; Cer, ceramide. Means and ±s.d. are shown (n=3). ***P<0.001; **P<0.01; *P<0.05 (unpairedt-test). (b) Percentage contribution of lipid classes to total lipid composition of wild-type and ΔgABCG2 stage IV gametocytes. Neutral lipids are shown in blue, FC in green and polar lipids in red. (c) PCA of the neutral lipid classes DAG, TAG and CE. Left: score plot showing grouping of three replicate analyses of wild-type (red) and ΔgABCG2 (blue) samples.x(PCA1) andy(PCA2) axes represent the principal components accounting for the greatest and second greatest variability, respectively. PCA loading plot indicating the contribution of individual lipid species towards the observed differences in the lipid classes DAG, TAG and CE between wild-type and ΔgABCG2 gametocytes. For clarity reasons, only the three most changed lipid species are labeled. (d) Wild-type and gABCG2-disrupted gametocytes labelled with neutral lipid stain. BF, bright field. Scale bar, 5 μm. Figure 4: Altered lipid composition in gABCG2-knockout parasites. ( a ) Lipid profile of gABCG2-disrupted trophozoite (ΔgABCG2-T) and stage IV gametocyte (ΔgABCG2-G) compared with wild type. T, trophozoite; G, gametocyte; PG, phosphatidylglycerol; PS, phosphatidylserine; Cer, ceramide. Means and ±s.d. are shown ( n =3). *** P <0.001; ** P <0.01; * P <0.05 (unpaired t -test). ( b ) Percentage contribution of lipid classes to total lipid composition of wild-type and ΔgABCG2 stage IV gametocytes. Neutral lipids are shown in blue, FC in green and polar lipids in red. ( c ) PCA of the neutral lipid classes DAG, TAG and CE. Left: score plot showing grouping of three replicate analyses of wild-type (red) and ΔgABCG2 (blue) samples. x (PCA1) and y (PCA2) axes represent the principal components accounting for the greatest and second greatest variability, respectively. PCA loading plot indicating the contribution of individual lipid species towards the observed differences in the lipid classes DAG, TAG and CE between wild-type and ΔgABCG2 gametocytes. For clarity reasons, only the three most changed lipid species are labeled. ( d ) Wild-type and gABCG2-disrupted gametocytes labelled with neutral lipid stain. BF, bright field. Scale bar, 5 μm. Full size image In gametocytes, the lipid composition of membranes is more complex and includes cholesteryl esters (CEs) and sphingomyelin (SM; Fig. 4a ). In this phase of the life cycle, FC and PC are the major lipids ( Fig. 4a,b ). A comparison of the lipid profiles of equivalent numbers of gametocyte-stage-parasitized erythrocytes from wild type to gABCG2-knockout cell lines revealed a significant increase in the amount of PE, which is the most abundant lipid in ΔgABCG2-infected erythrocytes. This is accompanied by a reduction in the neutral lipids CE, diacylglycerol (DAG) and triacylglycerol (TAG) in the ΔgABCG2-infected erythrocytes, compared with erythrocytes infected with wild-type parasites, where they together constitute 24% of the total lipid content ( Fig. 4b ). In addition, the gametocyte-stage ΔgABCG2-infected erythrocytes showed an increase in the amount of phosphatidylglycerol compared with erythrocytes infected with wild-type parasites. Although the level of FC was not altered, the ratio of cholesterol to phospholipids decreased significantly, from 0.62 in wild type to 0.37 in the ΔgABCG2-infected erythrocytes ( Supplementary Table 2 ). To identify individual lipid species that contribute in particular to the observed differences in the neutral lipids’ composition of wild-type and ΔgABCG2 gametocytes, we performed principal component analyses (PCA) for the lipid classes DAG, TAG and CE ( Fig. 4c ). For each lipid class, the three individual samples taken for the wild-type and knockout gametocytes aggregate in distinct clusters (left hand side scatter plot). The differences observed in DAG are due mainly to the ΔgABCG2 gametocytes having reduced levels of DAG species containing predominantly C18 acyl chains and having either a single, or no, double bond, for example, DAG 16:0_18:1, DAG 18:0_18:1, DAG 18:1_18:1. In the ΔgABCG2 gametocytes, DAG 18:1_20:5 and DAG 18:1_22:6 are the only neutral lipid species that are marginally increased relative to wild-type gametocytes. The three major lipid species that contribute to the observed reduction in TAG in the ΔgABCG2 gametocytes are 52:2, 50:2 and 50:1. For the CE, 18:2, 18:1 and 16:0 are the species that show a particular reduction in the ΔgABCG2 gametocytes relative to wild-type gametocytes. Lipid staining of ΔgABCG2 gametocytes indicated that the structure with which gABCG2 is associated in wild-type parasites is absent from the knockout line ( Fig. 4d ); however, in the absence of other specific markers for this lipid structure, it is difficult to draw definitive conclusions in this regard. Disruption of gABCG2 results in increased gametocyte formation On induction of gametocytogenesis, two independently derived clones of the ΔgABCG2 cell lines both consistently produced two to three times more gametocytes than the parental wild-type cell line ( Fig. 5a ). The increase in gametocyte numbers could be observed as early as gametocytes can be morphologically distinguished. The increase in gametocyte numbers also translated into increased numbers of gametes. 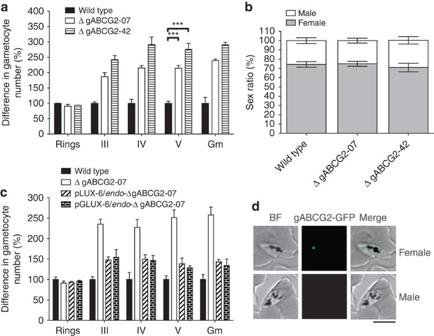Figure 5: gABCG2-knockout parasite lines show increased gametocyte production. (a) Numbers of RBCs infected with 3D7-wild-type and clonal-knockout (ΔgABCG2-07 and ΔgABCG2-42) parasites at different stages were counted using a flow cytometer. At least 1,000 infected RBCs per experiment were counted. Knockout parasite numbers relative to the wild-type numbers are shown. III–V, gametocytes stage 3 to stage 5. Gm, gametes. Means and ±s.d. of three independent experiments are shown. ***P<0.001 (unpairedt-test). (b) The sex ratio of gABCG2-07-disrupted parasites is unaltered. Mature male and female gametocytes of 3D7-wild-type and -knockout (ΔgABCG2-07 and ΔgABCG2-42) cell lines were differentiated using morphological characteristics of mature gametocytes in Giemsa-stained thin smears69. At least 500 gametocytes per experiment were counted by two independent microscopists from de-identified samples. Means and ±s.d. of three independent experiments are shown. (c) Expression of gABCG2 under the control of the endogenous promoter results in gametocyte production reverting to close to that in wild-type parasites. The numbers of RBCs infected with 3D7-wild-type, -knockout ΔgABCG2-07, untagged endogenous complementation (pLUX-6/endo-ΔPfgABCG2-07) and GFP-tagged endogenous complementation (pGLUX-6/endo-ΔPfgABCG2-07) parasites at different stages were counted by flow cytometer. At least 1,000 infected RBCs per experiment were counted. Transgenic parasite numbers relative to the wild-type numbers are shown. III–V, gametocytes stage 3 to stage 5. Gm, gametes. Means and ±s.d. of three independent experiments are shown. (d) Live-cell fluorescence microscopy of pGLUX-6/endo-ΔPfgABCG2-07 transfectant was performed on late-stage gametocyte. BF, bright field. Scale bar, 5 μm. Figure 5: gABCG2-knockout parasite lines show increased gametocyte production. ( a ) Numbers of RBCs infected with 3D7-wild-type and clonal-knockout (ΔgABCG2-07 and ΔgABCG2-42) parasites at different stages were counted using a flow cytometer. At least 1,000 infected RBCs per experiment were counted. Knockout parasite numbers relative to the wild-type numbers are shown. III–V, gametocytes stage 3 to stage 5. Gm, gametes. Means and ±s.d. of three independent experiments are shown. *** P <0.001 (unpaired t -test). ( b ) The sex ratio of gABCG2-07-disrupted parasites is unaltered. Mature male and female gametocytes of 3D7-wild-type and -knockout (ΔgABCG2-07 and ΔgABCG2-42) cell lines were differentiated using morphological characteristics of mature gametocytes in Giemsa-stained thin smears [69] . At least 500 gametocytes per experiment were counted by two independent microscopists from de-identified samples. Means and ±s.d. of three independent experiments are shown. ( c ) Expression of gABCG2 under the control of the endogenous promoter results in gametocyte production reverting to close to that in wild-type parasites. The numbers of RBCs infected with 3D7-wild-type, -knockout ΔgABCG2-07, untagged endogenous complementation (pLUX-6/ endo -ΔPfgABCG2-07) and GFP-tagged endogenous complementation (pGLUX-6/ endo -ΔPfgABCG2-07) parasites at different stages were counted by flow cytometer. At least 1,000 infected RBCs per experiment were counted. Transgenic parasite numbers relative to the wild-type numbers are shown. III–V, gametocytes stage 3 to stage 5. Gm, gametes. Means and ±s.d. of three independent experiments are shown. ( d ) Live-cell fluorescence microscopy of pGLUX-6/ endo -ΔPfgABCG2-07 transfectant was performed on late-stage gametocyte. BF, bright field. Scale bar, 5 μm. Full size image Despite the gender-specific nature of gABCG2 expression, the proportion of male to female gametocytes formed by the ΔgABCG2 parasites was not significantly different from that formed by the wild-type parents; the male to female ratio was 1:3 in both cases ( Fig. 5b ), matching previous reports [22] . To complement the phenotype of increased gametocyte production in ΔgABCG2 cells, we cloned a plasmid in which gABCG2 expression was placed under the control of the 1 kb region immediately upstream of the start codon of the gABCG2 gene ( Supplementary Fig. 5A ). This plasmid was transfected into ΔgABCG2 cells and the resulting cell line was analysed for the ability to form gametocytes ( Fig. 5c ). Gametocyte numbers were significantly reduced compared with the knockout lines and were only slightly higher than those observed in parental wild-type cells ( Fig. 5c —striped bars). This complementation confirms that the altered phenotype in gABCG2-knockout cells may be attributed to the lack of gABCG2 in these cells, rather than to other, atopic, effects. We also constructed a plasmid with the 1 kb upstream region driving the expression of c-terminally GFP-tagged gABCG2 ( Supplementary Fig. 5B ). Expression of the chimeric gABCG2-GFP protein complemented the ΔgABCG2 phenotype to the same level as untagged gABCG2 ( Fig. 5c —brick bars). GFP fluorescence was restricted to female gametocytes only and was observed as a single dot, similar to the structure seen in endogenously tagged gABCG2-GFP cell lines ( Fig. 5d ). Together, these results indicate that the altered phenotype observed in the ΔgABCG2 cells can be specifically attributed to the absence of gABCG2 and that the c-terminal GFP tag does not interfere with the function of gABCG2. Elevated cGMP levels in ΔgABCG2 trophozoites Secondary messengers such as DAG, cyclic adenosine monophosphate (cAMP) and cyclic guanyl monophosphate (cGMP) have been implicated in the commitment, differentiation and development of sexual forms of Plasmodium (see ref. 2 for review). A comparison of cAMP levels in trophozoites stages of wild-type and ΔgABCG2-infected erythrocytes revealed no significant difference in cAMP levels ( Fig. 6 ) between the two lines. By contrast, cGMP levels increased by 70% in erythrocytes infected with ΔgABCG2 trophozoite-stage parasites, relative to those infected with wild-type trophozoites. 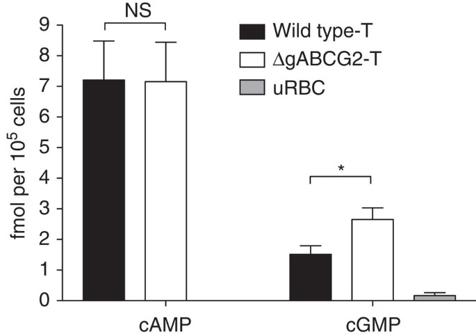Figure 6: ΔgABCG2 trophozoite parasites produce more cGMP than their wild-type counterparts. cAMP and cGMP levels in ΔgABCG2-disrupted trophozoites (T) were compared with those in wild-type trophozoites. Means and s.d. are shown (n=3). The data were compared using unpairedt-test. NS, not significant; uRBC, uninfected RBC; *P<0.05. Figure 6: ΔgABCG2 trophozoite parasites produce more cGMP than their wild-type counterparts. cAMP and cGMP levels in ΔgABCG2-disrupted trophozoites (T) were compared with those in wild-type trophozoites. Means and s.d. are shown ( n =3). The data were compared using unpaired t -test. NS, not significant; uRBC, uninfected RBC; * P <0.05. Full size image gABCG2 expression under CRT promoter renders it non-functional To explore the influence of the endogenous promoter on the localization and sex-specific expression of gABCG2, we cloned the coding region of gABCG2 into the pGLUX-6 vector ( Supplementary Fig. 5C ) [23] and transfected this construct into ΔgABCG2 cells to express episomally a GFP-tagged version of gABCG2 under the control of the promoter for the chloroquine resistance transporter gene ( CRT ). The CRT protein is expressed in the asexual stages of the parasite life cycle, with expression reaching a maximum in late ring stages [24] , and localizes to the DV membrane [25] . In the cell lines expressing gABCG2-GFP under the control of the CRT promoter, green fluorescence was observed at all stages of the intraerythrocytic life cycle ( Fig. 7a ). In early rings, the fluorescence pattern reveals two dots connected by a thin band near the nucleus—a pattern that is reminiscent of endoplasmic reticulum [26] . In late trophozoites, the chimeric protein was localized close to the DV. 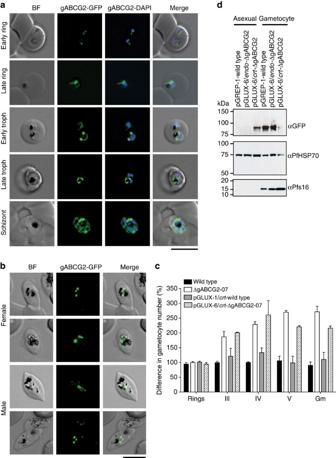Figure 7: Expression of gABCG2 under the control of the CRT promoter in ΔgABCG2 parasites does not reverse gametocyte overproduction. Live-cell fluorescence microscopy of pGLUX-6/crt-ΔPfgABCG2 transfectant was performed at asexual (a) and gametocyte (b) stages. BF, bright field. Scale bar, 5 μm. (c) The numbers of RBCs infected with 3D7-wild-type, -knockout (ΔgABCG2-07), overexpression (pGLUX-1/crt-wild type) and CRT complementation (pGLUX-6/crt-ΔPfgABCG2-07) parasites at different stages were counted by flow cytometer. At least 1,000 infected RBCs per experiment were counted. Transgenic parasite numbers relative to the wild-type numbers are shown. III–V, gametocytes stage 3 to stage 5. Gm, gametes. Means (±s.d.) are shown (n=3). (d) The expression of gABCG2 was determined by western blot performed on the synchronous GFP-tagged gABCG2 (pGREP-1-wild type), GFP-tagged endogenous complement (pGLUX-6/endo-ΔPfgABCG2) and GFP-tagged CRT complement (pGLUX-6/crt-ΔPfgABCG2) parasite samples using anti-GFP antibody. The membranes were also probed with anti-PfHSP70 antibody as a loading control. Antibody against Pfs16 was used as a marker of gametocytes. For full-sized western blots, seeSupplementary Fig. 8. Figure 7: Expression of gABCG2 under the control of the CRT promoter in ΔgABCG2 parasites does not reverse gametocyte overproduction. Live-cell fluorescence microscopy of pGLUX-6/ crt -ΔPfgABCG2 transfectant was performed at asexual ( a ) and gametocyte ( b ) stages. BF, bright field. Scale bar, 5 μm. ( c ) The numbers of RBCs infected with 3D7-wild-type, -knockout (ΔgABCG2-07), overexpression (pGLUX-1/ crt -wild type) and CRT complementation (pGLUX-6/ crt -ΔPfgABCG2-07) parasites at different stages were counted by flow cytometer. At least 1,000 infected RBCs per experiment were counted. Transgenic parasite numbers relative to the wild-type numbers are shown. III–V, gametocytes stage 3 to stage 5. Gm, gametes. Means (±s.d.) are shown ( n =3). ( d ) The expression of gABCG2 was determined by western blot performed on the synchronous GFP-tagged gABCG2 (pGREP-1-wild type), GFP-tagged endogenous complement (pGLUX-6/ endo -ΔPfgABCG2) and GFP-tagged CRT complement (pGLUX-6/ crt -ΔPfgABCG2) parasite samples using anti-GFP antibody. The membranes were also probed with anti-PfHSP70 antibody as a loading control. Antibody against Pfs16 was used as a marker of gametocytes. For full-sized western blots, see Supplementary Fig. 8 . Full size image This localization in asexual stages could either be due to a specific functional targeting to the DV or to gABCG2 being sent to the DV for degradation. Several reports describe nonspecific delivery of GFP-tagged proteins to the DV arising as a result of inappropriate timing of expression and/or absence of the appropriate target organelle [27] , [28] . In gametocytes, the fluorescence emanating from the protein expressed under the control of the CRT promoter was observed as several distinct spots near the hemozoin crystals, consistent with localization in the DV membrane ( Fig. 7b ). Expression of gABCG2 under the control of the CRT promoter also abolished the restriction of expression to female gametocytes, with the chimeric protein now observed in both male and female gametocytes ( Fig. 7b ). We also analysed the effect of gABCG2 overexpression on the number of gametocytes produced ( Fig. 7c ). Transfection of wild-type cells with the plasmid pGLUX-1/crt- PfgABCG2 ( Supplementary Fig. 6A , for full-sized western blots, see Supplementary Fig. 9 ), resulting in the expression of gABCG2-GFP on top of the expression of endogenous gABCG2, had no significant effect on the formation of sexual-stage parasites; gametocyte numbers remained at wild-type level (light grey bars), with an ~3:1 female to male ratio ( Supplementary Fig. 10 ). When a similar construct, encoding gABCG2-GFP under the control of the CRT promoter, was made in the pGLUX-6 vector (pGLUX-6 being a derivative of pGLUX-1 (ref. 23 ), where the selectable marker human dihydrofolate reductase (hDHFR) was replaced by puromycin acetyl transferase; Mikkonen and Maier, manuscript in preparation; Supplementary Fig. 5C ) and was transfected into the ΔgABCG2 cells, the wild-type level of gametocytes was not restored ( Fig. 7c , dotted bars). Using western blot, we compared the expression level and timing of the episomal expression of gABCG2 under the control of the two different promoters in the ΔgABCG2 background ( Fig. 7d ). As expected, the CRT promoter led to a significant expression of gABCG2 in asexual stages, whereas the expression level in gametocytes was very low. This provides an explanation for the inability of this construct to restore gametocyte production levels in ΔgABCG2 cells to those seen in wild-type cells. In contrast, placing gABCG2 under the control of the region upstream of the translation start site of gABCG2 containing the native promoter resulted in stage-specific expression of the protein in gametocytes ( Fig. 7d ). Together, the data indicate that gABCG2-GFP expressed under the CRT promoter is unable to restore the function of gABCG2 in the ΔgABCG2 cells. This highlights the importance of the promoter for the correct localization, expression level, female-specific expression and function of the protein. The ABCG family member gABCG2 is expressed predominantly in the sexual, gametocyte phase of the malaria parasite life cycle. Low-level expression was also detected in young ‘ring-stage’ asexual parasites but not in the more mature asexual forms. Expression in sexual-stage parasites is limited to female gametocytes, with the protein localizing to a novel, neutral lipid-rich structure. Deletion of the gene encoding the protein decreased the amount of neutral lipids detected in gametocyte-infected erythrocytes, as well as increasing the number of gametocytes formed by some threefold. ABCG proteins in other systems function either as homodimers or heterodimers, and are known to transport a diverse range of substrates, including lipids [4] . In the malaria parasite, each parasite stage displays a distinct lipid profile [29] , reflecting different requirements for membrane biogenesis, energy and signalling. A possible interpretation of the results obtained here is that gABCG2 functions to transport neutral lipids into the structure to which the protein localizes in the female gametocyte, and that this structure thereby serves as a neutral lipid storage compartment. In the absence of the protein, the parasite is unable to sequester neutral lipids into this compartment and the total neutral lipid content therefore decreases. Neutral lipids are required to support membrane biogenesis, and are also known to play a role in the phenomenon of haemozoin formation in the malaria parasite’s DV [30] . ABCG2, in mammals, protects against toxic levels of the haeme precursor protoporphyrin IX (ref. 31 ) and ABCG2-deficient rodent cells show increased sensitivity to hypoxic conditions, due to the accumulation of cellular haeme metabolites [32] . The malaria parasite detoxifies the same metabolites through haemozoin formation in the DV [33] ; however, the gABCG2 protein is not expressed in mature asexual-stage parasites, in which haemoglobin digestion occurs. Instead, gABCG2 appears to have an effect on maintaining asexual propagation, since a higher proportion of parasites commit to sexual differentiation in the absence of gABCG2. In this context, it is interesting to note that the unknown lipid-rich structure observed in female gametocytes is, at least in early-stage gametocytes, close to the DV. The fact that this single structure moves towards one apical end of the gametocyte might indicate a polarized organization of the gametocyte in general. The single, female-specific, neutral lipid-rich structure could not be linked to any known cellular organelle in P. falciparum . However, its composition, localization and appearance are reminiscent of lipid bodies. Lipid bodies (that is, deposits of neutral lipids surrounded by a phospholipid monolayer and numerous proteins) are present in both prokaryotic and eukaryotic cells and play a major role in lipid homeostasis, protection from lipotoxicity, energy storage, signalling and membrane trafficking [34] . Lipid bodies can be induced in response to environmental changes or stress [35] . They have been described previously in P. falciparum but thus far this has been restricted to asexual-stage parasites, which contain neutral lipid bodies that range from >1 to 2 μm in diameter and that are closely associated with the DV. It has been suggested that lipid bodies in Plasmodium are derived from the digestion of phospholipid-containing transport vesicles [29] . Their relative abundance and localization in asexual forms is stage dependent [29] , and such structures have not previously been investigated in sexual-stage parasites. The major lipid species stored in the lipid bodies of mature asexual parasite stages are DAG and TAG [36] . Both lipid classes are significantly elevated in asexual P. falciparum -infected erythrocytes relative to uninfected erythrocytes [36] . In mammalian and yeast cells, lipid bodies consist of a neutral lipid core surrounded by a monolayer of phospholipids (mainly PC and PE) and proteins [37] . In ABCG2-deficient gametocytes, the levels of lipids that are typically found in the core of lipid bodies (CEs, TAG and DAG) are decreased, whereas the level of the lipid that typically surrounds the core, PE, is increased. No ABCG2 transporter is known to be associated with lipid bodies. However, ABCG2 proteins have been shown to be present both on the plasma membrane and on intracellular membranes of human cancer cells and cells of the Drosophila compound eye [38] , [39] . Potential mechanisms by which proteins that are normally located in the lipid bilayer of plasma membranes may relocate to the monolayer of lipid bodies have been suggested previously [34] . It would therefore seem plausible that the gABCG2-containing structure rich in neutral lipids might represent a specialized form of lipid body. One possible function of the gABCG2-containing, lipid body-like structures in female gametocytes is to prepare the parasite for the transition from the human environment to the conditions encountered in the mosquito, serving to sequester lipids from the human host that are less readily available in the mosquito host. For example, neither insect host nor Plasmodium parasite are able to synthesize cholesterol de novo , but parasites rely on the presence of cholesterol [40] , [41] . Both FC and the biologically inert storage form, CEs, are reduced in ΔgABCG2-infected red blood cells (RBCs). Alternatively, similar to the stockpiling of mRNA for use after gametogenesis [42] , neutral lipids could be accumulated for rapid utilization in the transition from gametes to zygote. The lipid body-like structure could also serve as a ‘buffer’ organelle: TAG is a major lipid component of the insect diet, but is rapidly absorbed from the midgut [43] . In the haemolymph of the mosquito, TAG is bound to lipophorin potentially rendering it inaccessible to the parasite [44] . In addition, significant amounts of neutral lipids are required during egg production in female mosquitoes [45] . Hence, it is conceivable that the amount of neutral lipids available to the parasite inside the mosquito fluctuates significantly and that the observed accumulation of neutral lipids might represent a mechanism to ensure a constant and reliable supply of neutral lipids. Female gametes contribute virtually all cellular material to the newly formed zygotes and, subsequently, the ookinetes in the insect host, whereas the contribution of the male gametocytes is mainly in the form of genetic material. Therefore, the female-specific expression of gABCG2 would fit with the protein playing a role in sequestering essential lipids from the human host, for use in the insect stage(s). The observation that disrupting the gene encoding gABCG2 leads to a threefold increase in the number of gametocytes generated (while not perturbing the relative proportions of males and females) raises the possibility that the protein plays a role in the phenomenon of commitment to gametocytogenesis. The gABCG2 protein is expressed at low levels at the ring stage and it is presumably the loss of expression at this stage in the knockout line that gives rise to the increased gametocyte production. The process of commitment in P. falciparum is thought to occur at the schizont stage of intraerythrocytic development [2] , however, there are also reports that place the period of sensitivity for gametocyte commitment around the time of invasion [46] . How the loss of the protein at the ring stage might have this effect is unclear. Gametocytogenesis is induced under conditions of stress (for example, over-crowding; presence of immune pressure, hormones, drugs; ref. 2 ) and one possibility is that the increase in gametocyte numbers seen here in the ΔgABCG2 parasites is a response to a general (as yet unidentified) stress resulting from the loss of the protein from ring-stage parasites. The observation that the deletion of the female-specific gABCG2 results in more gametocytes, but no shift in the sex ratio, together with the fact that the progeny of an individual sexually committed schizont forms either male or female gametocytes only [47] suggests two independent mechanisms for the regulation of gametocyte commitment and sex differentiation. However, another possibility is that the protein plays a more specific role in suppressing gametocytogenesis in wild-type parasites, with the suppression lifted in the knockout strains. This would mean that gABCG2 might have two different functions depending on the developmental stage: a role in the commitment process in ring-stage parasite and a second, distinct role in lipid segregation and accumulation in gametocytes. Induction of gametocytogenesis is known to involve second messenger molecules such as cAMP [48] . No significant changes in cAMP levels were observed in the trophozoite stage of ΔgABCG2 parasites; however there was a significant increase in cGMP levels. cGMP has been implicated in the early stages of P. falciparum gametocyte activation and in the development of sexual forms of the parasite in insects [49] , raising the possibility that the effect of gABCG2 on cGMP levels might play a role in the observed increase in gametocyte numbers. It is perhaps relevant to note that cGMP has been found to be a substrate for ABCG2 in other organisms: in mice, ABCG2 transports cGMP into erythrocyte vesicles playing a role in cGMP secretion [50] and in Drosophila ABCG2 transports cGMP in the malpighian tubules [51] . This raises the possibility that cGMP is a substrate for gABCG2 and that the increased cGMP levels might be a consequence of a cGMP transport defect. If gABCG2 does play a role in commitment, this must be in asexual-stage parasites. The observation that gABCG2 is expressed in early ring-stage parasites is consistent with this notion ( Fig. 1b,c ), although perhaps at odds with the previous report that cells are most sensitive to commitment signals in the late troph/schizont stage [2] . The possibility that gABCG2 performs different roles, and perhaps transports different substrates, at different life stages is not without precedent. In Drosophila , ABCG2 plays a role in the transport of eye pigment precursor in the larva and pupa [52] . In adults, however, the protein is located on vesicle in the malpighian tubules, where it is implicated in the sequestration and transport of cGMP across the Malpighian tubule [51] . Substrate specificity is regulated by interactions between different sets of ‘half-transporter’ molecules and/or multiple pharmacologically distinct substrate-binding sites [53] . In a recent publication, Eastman et al. [54] investigated the involvement of gABCG2 in drug transport and drug resistance in gametocytes. In this study, the gene for gABCG2 was also deleted, but in contrast to our findings, there was a decrease in gametocyte production following removal of gABCG2. In this earlier study, the two gene-deletion clones analysed were derived from a single transfection, and in their discussion the authors pointed out that a secondary off-target effect responsible for the decrease in gametocyte numbers cannot be excluded. Several attempts to restore gametocyte production by complementing the gene were unsuccessful [54] . Hence, the two principal criteria for an experimental genetics analysis [55] were not met, making it difficult to reconcile the apparent discrepancies to our findings. Using gABCG2 as a target gene, we provide a conclusive example that a detailed characterization using P. falciparum clones from independent transfections and complete recovery of the observed defects on complementation under the endogenous, but not from a heterologous, promoter is possible. The female-specific expression of gABCG2 raises the possibility that it might be exploited as a research tool. Gender-specific markers are sparse, and differentiating between male and female P. falciparum gametocyte populations has been reliant on differentially expressed genes (for example, Pfg377 for females and alpha tubulin II for males; refs 56 , 57 ) leading to conflicting results sometimes [58] . gABCG2 is, to our knowledge, the first exclusively female-specific marker in P. falciparum and, hence, holds great promise as a tool to identify and isolate female P. falciparum gametocytes, perhaps during the first hours of commitment to gametocytogenesis. We have shown that the promoter activity is responsible for the female-specific expression and further studies are warranted to explore the molecular mechanism underlying this sex-specific control of gene expression. In serving as a sex-specific marker, gABCG2 will facilitate further studies designed to shine new light on a crucial, yet enigmatic, part of the malaria parasite life cycle. DNA constructs Annotated sequence data were obtained from PlasmoDB ( http://www.plasmodb.org/ ). To tag gABCG2 with GFP at the carboxy terminus, a PfgABCG2 fragment (nucleotide (nt) 1,113–1,979 of the PF14_0244 gene sequence) was amplified from P. falciparum 3D7 genomic DNA with primers al116/al117 ( Supplementary Table 1 ), and cloned into pGREP-1 (ref. 23 ) (a vector for GFP tagging of protein expressed from the endogenous locus; restriction sites used SacII and XhoI) to produce pGREP-1/PfgABCG2 ( Supplementary Fig. 2A ). To disrupt gABCG2 , a 5′ fragment and 3′ fragment of the gABCG2 locus were amplified using primers al112/al113 and al114/al115 and cloned into pCC-1 vector [21] (a vector to generate gene knockouts via double recombination) at SacII/SpeI and EcoRI/AvrII sites to generate the pCC-1/ PfgABCG2 construct ( Supplementary Fig. 4A ). To create an asexual gABCG2 overexpression cell line, the full-length PfgABCG2 region was amplified with primers al118/al119 and cloned into the pGLUX-1 vector [23] (a vector to express GFP-fusion proteins episomally; restriction sites used: XhoI and KpnI) to generate pGLUX-1/ crt - PfgABCG2 vector under the CRT (chloroquine resistance transporter) promoter control for episomal expression ( Supplementary Fig. 6A ). For complementation, the hDHFR drug selection cassette from the vector pGLUX-1/ crt - PfgABCG2 was replaced by the puromycin acetyl transferase drug selection cassette to generate the pGLUX-6/ crt - PfgABCG2 vector (Mikkonen and Maier, manuscript in preparation; Supplementary Fig. 5C ). Here, gABCG2 expression is driven by the CRT promoter. Subsequently, the vector pGLUX-6/ crt - gABCG2 was modified by replacing the CRT promoter with the gABCG2 endogenous promoter (1,084 nt upstream, primers al240/al241) to generate pGLUX-6/ endo / PfgABCG2-GFP vector (with GFP tag) and pGLUX-6/ endo / PfgABCG2 (without GFP tag; Supplementary Fig. 5A and B ). In these plasmids, gABCG2 expression is driven by the endogenous promoter. All the inserted DNA regions were sequenced to verify the gene sequences and the insertions. For parasite transfection, all plasmids were purified using a Purelink maxiprep kit (Invitrogen). Parasite culture and transfection P. falciparum 3D7 parasites were cultured using standard methods with slight modifications [59] . Briefly, parasites were maintained in O+ RBCs at 4% haematocrit resuspended in RPMI medium supplemented with 10 mM glucose, 480 μM hypoxanthine, 20 μg ml −1 gentamycin, 2.5% (v/v) human serum and 0.75% (w/v) Albumax II. Cultures were maintained at 37 °C under microaerophilic conditions (1% O 2 , 5% CO 2 , 94% N 2 ). Two days before transfection, ring-stage parasites were synchronized by 5% sorbitol treatment. Highly synchronous trophozoites were obtained on the following day and split into 1% parasitemia. On the next day, transfections were done by electroporation of 100 μg of plasmid DNA into >5% synchronized ring-stage parasites using an established procedure [23] . For pGREP-1, pGLUX-1 and pCC-1, parasites were selected with 2 nM WR99210 (Jacobus Pharmaceuticals) and weekly replenishment of fresh RBCs for about 4 weeks or until resistant parasites appeared [23] . Parasites containing integrated forms of the constructs were enriched using drug on–off cycles. DNA from 3D7 parental and all transfected parasite lines were purified using the DNeasy blood and tissue kit (Qiagen) as per the manufacturer’s instructions and screened by Southern blot using a standard protocol to detect plasmid integration into the gABCG2 locus [23] . Single clones of two independent gABCG2-knockout transfections were obtained by limited dilution. Two knockout clones were selected on a random basis for phenotypic analysis. To complement the gABCG2 disruption mutants, pGLUX-6/ crt - gABCG2 (under CRT promoter control) and pGLUX-6/ endo / PfgABCG2 (under endogenous promoter control) were transfected into a gABCG2-knockout clone (ΔgABCG2-07) and selected with 100 pg μl −1 puromycin and 2 nM WR99210 until resistant parasites appeared. The expression of the tagged protein was confirmed by western blot using mouse anti-GFP antibodies (clone 7.1 and 13.1, Roche, 1:1,000). Gametocyte commitment and harvesting Induction of gametocytogenesis was performed as described previously [60] with slight modifications. Briefly, 2% synchronous trophozoites were incubated overnight to obtain about 8% ring-stage parasites. The culture was stressed by replacing 75% of the spent medium with fresh medium. On the next day (designated as day −1), when parasites reached trophozoite stage, the culture was split to obtain 2% trophozoites with the retention of one-third of the spent medium. After overnight incubation, about 8% ‘stressed’ ring-stage parasites appeared in the culture on the next day, which was designated as day 0. All the ring-stage parasites were magnet purified and adjusted to 2% parasitemia. Subsequently, the medium was changed daily with fresh medium containing 50 mM GluNAc to prevent non-committed asexual stages from propagating [61] and the culture was maintained for 12 days until mature gametocytes were observed to be present. Gametocytaemia was determined by counting 200,000 total RBCs by flow cytometer using 1 μM SYTO16 (Invitrogen) to detect the parasite’s nucleic acids. After this stress-induced commitment, specific stage gametocytes were collected every 2 days by magnet purification. Mature male and female gametocytes were distinguished from one another on the basis of the morphological characteristics of mature gametocytes in Giemsa-stained thin smears [2] . The sex ratio of male to female gametocytes was determined by counting at least 500 gametocytes on each slide. Indirect immunofluorescence assay Parasites were allowed to adhere to concanavalin A-coated slides for 15 min, then fixed in 2% v/v paraformaldehyde/0.008% glutaraldehyde for 20 min and washed with phosphate buffered saline (PBS), before being permeabilized in 0.1% w/v Triton X-100 (Sigma) for 10 min. After being incubated in diluted primary antibodies in 3% w/v bovine serum albumin/PBS for at least 2 h, the cells were then washed in PBS. Primary antibodies used were: mouse anti-GFP (1:1,000, Roche), rabbit anti-GFP (1:1,000; a gift from M. Ryan, La Trobe University), rabbit anti-ACP (1:1,000; a gift from G. McFadden, the University of Melbourne), rabbit anti-BET3 (1:1,000; a gift from L. Tilley, the University of Melbourne), mouse anti-Pfg377 (1:500; a gift from Pietro Alano, Istituto Superiore di Sanita Roma) and MitoTracker (1:2,000, Invitrogen). The cells were then incubated with secondary antibodies conjugated to either Alexa Fluor 488 (green) or 594 (red) dyes (Invitrogen), for at least 1 h, then mounted in Vectashield containing DAPI (4′,6-diamidino-2-phenylindole) and examined with a restorative widefield deconvolution microscope (DeltaVision Elite, Applied Precision) using a × 100 objective (1.4 NA). Images displayed are maximum projection images of whole cell z stacks (taken at intervals of 0.2 μm). Images were deconvolved using the softWoRx acquisition software (version 5.0) and then processed with ImageJ 1.43u software (NIH, USA). Colour, brightness and contrast were modified for clarity. SDS–PAGE analysis and western blot Synchronous parasites were enriched using magnetic cell-sorting columns (CS and D columns; MACS Cell Separation, Miltenyi Biotec) and RBC membrane was lysed by incubating parasites on ice with 0.15% w/v saponin solution for 15 min. Then, parasites were pelleted and washed in PBS containing Complete Protease Inhibitor Cocktail (Roche) until the supernatant colour was clear. The parasite pellets were either stored at −70 °C or immediately treated with 2.5 U benzonase nuclease (Novagen) per 60 μl pellet and taken up in lithium dodecyl sulfate (LDS) sample buffer (Invitrogen, Life Technologies) containing 10% 2-mercaptoethanol (Sigma). Denatured proteins were separated on 4–12% Bis-Tris NuPAGE gels (Invitrogen, Life Technologies). The proteins were transferred to a nitrocellulose membrane using the iBlot system (Invitrogen, Life Technologies) according to the manufacturer’s instructions. Following the transfer, the membranes were blocked with PBS solution containing 10% milk powder. Both primary and secondary antibodies were made up in PBS containing 1% milk powder. Primary antibodies used were: rabbit anti-GFP (1:1,000), mouse anti-PfHSP70 (1:1,000; ref. 21 ) and mouse anti-Pfs16 (1:1,000; Supplementary Methods ). Horseradish peroxidase-coupled goat anti-mouse IgG (1:2,000; Southern Biotech) or donkey anti-rabbit IgG (1:5,000; GE Healthcare) were used as secondary antibodies. Relative mRNA level quantification The wild-type ring-stage P. falciparum 3D7 parasites were highly synchronised by 4-h double sorbitol treatment. Asexual rings, trophozoites and schizonts were then collected 8 h apart, while highly synchronous stage IV gametocytes were obtained at day 8 of commitment (gametocyte commitment and harvesting procedure). Total RNA was isolated using an RNeasy mini kit (Qiagen) and first-strand complementary DNA was prepared with a QuantiTect reverse transcription kit (Qiagen) according to the manufacturer’s instructions. The wild-type parasite genomic DNA was isolated with the DNeasy blood & tissue kit (Qiagen) and used as template for the standard curve. For the hydrolysis probe-based real-time PCR, primer and probe sets ( Supplementary Table 2 ) were designed and generated by Integrated DNA Technologies for PF14_0244 and reference gene PFL2215w (ActinI, which is relatively equally expressed in all parasite stages [62] ). The assay was performed with a Light Cycler 480 (Roche) to detect gABCG2 mRNA amplification in the 6-carboxyfluorescein (FAM) channel and reference actin mRNA amplification in the hexachlorofluorescein (HEX) channel concurrently in the same reaction. The original mRNA copy number of both genes was then calculated based on the standard curve established with serial dilutions of genomic DNA. The relative expression levels of gABCG2 in different parasite stages were compared using mRNA copy number of PF14_0244 normalized to that of PFL2215w (ref. 62 ). All experiments were performed in three independent replicates. Lipid labelling assay Neutral and polar lipid labelling were performed according to the manufacturer’s instructions. Briefly, parasites were washed three times with PBS before being fixed with 4% v/v formaldehyde in PBS for 20 min at room temperature. The cells were then washed three times with PBS and incubated with LipidTOX Red neutral lipid stain (1:200 in PBS; Invitrogen), Nile red (1 μg ml −1 in PBS; Sigma) or BODIPY-TR-ceramide (0.7 μmol l −1 ; Invitrogen) at room temperature for 30 min. The cells were then washed three times with PBS before being imaged with a filter set for Alexa Fluor 594 dye on a deconvolution microscope (DeltaVision Elite, Applied Precision) or three-dimensional structured illumination microscope (3D-SIM; DeltaVision OMX OMX V4, GE/Applied Precision). A combination of InsightSSI Solid State Illumination and light-emitting diode transillumination light sources, a high-speed shuttering system and a Cascade EM camera, were used to image the cells at the × 100 objective. Images were deconvolved using the softWoRx acquisition software (version 5.0) with the Wiener filter setting and then post-processed with ImageJ 1.43u software (NIH, USA). 3D-SIM [63] was performed on a DeltaVision OMX V4 (GE/Applied Precision) equipped with a × 60 Olympus UPlanSApo 1.42 NA oil immersion lens and sCMOS cameras (PCO AG). Samples were excited using 488 or 568 nm lasers and imaged using 528/48 and 609/37 nm band pass filters. All fluorescence images were processed using the Applied Precision SoftWoRx 6.1 software or Image J software ( http://rsbweb.nih.gov./ij/ ). Colour, brightness and contrast were modified for clarity. Lipidomic profile analysis by MS Each analysis was performed on three independent biological samples. Synchronous infected RBCs were enriched using magnetic cell-sorting columns (CS and D columns; MACS Cell Separation, Miltenyi Biotec), washed in PBS and then counted on a haemocytometer. Lipid extraction was performed using a modification of the method of Matyash et al. [64] In brief, 10 7 magnet-purified cells were added to 2 ml tough tubes (Geneworks, Hindmarsh, SA, Australia) on dry ice, fixed with 300 μl of methanol and stored at −80 °C until extraction step. An aliquot of 100 μl of methanol containing 0.01% butylated hydroxytoluene and internal standards (listed in Supplementary Table 3 ) was added to each tube. Samples were homogenized using a bead homogeniser (FastPrep-24, MP Biomedical, Seven Hills, NSW, Australia) at 6 m s −1 for 40 s and the homogenate removed to 2 ml microcentrifuge tubes (Eppendorf, North Ryde, NSW, Australia). Beads were washed with 100 μl of methanol and the wash added to the homogenate. A 1-ml aliquot of methyl-tert butyl ether was added and samples were vortexed at 4 °C for 1 h. A total of 300 μl of 150 mM ammonium acetate (liquid chromatography–MS grade, Fluka, Castle Hill, NSW, Australia) was added to induce phase separation. Tubes were vortexed for 15 min and centrifuged at 2,000 g for 5 min to complete phase separation. Approximately 800 μl of the upper organic layer was removed to a new 2 ml glass vial and stored at −20 °C until analysis. Extracts were diluted 40-fold into methanol:chloroform (2:1 v/v) containing 5 mM ammonium acetate before MS analysis. Mass spectra were acquired using a chip-based nanoESI source (TriVersa Nanomate, Advion, Ithaca, NY, USA) coupled to a hybrid linear ion-trap-triple quadrupole MS (QTRAP 5500, ABSCIEX, Foster City, CA, USA). A 10-μl aliquot of methanol:chloroform-diluted extract was aspirated from a sealed 96-well plate (Eppendorf Twin-Tec) and delivered into the MS via a nanoESI chip with an orifice diameter of 4.1 μm. The delivery gas was N 2 at a pressure of 0.4 p.s.i. and a spray voltage of ±1.15 kV was used for positive-ion acquisition. Target lipids and MS scan parameters are shown in Supplementary Table 4 . Experimental conditions for positive- and negative-ion mode acquisition were a declustering potential of ±100 V, entrance potential of ±10 V and a scan rate of 200 m/z U s −1 . Mass spectra were averaged over 50 scans. The mass spectrometry raw data of the lipidomics experiments have been deposited in the MetaboLights database with accession code MTBLS98 ( http://www.ebi.ac.uk/metabolights ). Data were analysed with LipidView (ABSCIEX) software version 1.2, including smoothing, identification, removal of isotope contribution from lower mass species and correction for isotope distribution. Ionized lipids detected with a signal-to-noise ratio (s/n) over 20 were included in the analysis. Extraction and solvent blanks were included in the analysis to allow exclusion of ions detected at lipid masses that result from extraction chemical or solvent impurities. Quantification was achieved in LipidView software by comparison of the peak area of individual lipids to their class-specific internal standards after isotope correction. Ions detected at masses that could be assigned to odd-chain fatty acid phospholipids or ether-linked phospholipids were assumed to be ether linked. Ether-linked PE species produce the 141 head group fragment at ~29%, the efficiency of diacyl PE species [65] ; therefore, a correction factor of 3.45 was applied to all ether–PE species [66] . SM species were detected using the 184.1 m/z precursor-ion scan, which cannot distinguish between isobaric dihydrosphingomyelin (DHSM) and SM species. Ions detected at masses that could be assigned to DHSM or SM were assumed to contain the major SM backbone d18:1, and are listed as species indicating the respective N-linked fatty acid. Lipid molecular species are notated in accordance with recently proposed shorthand by Liebisch et al. [67] (except for DAG and TAG). PCA data processing was performed using MarkerView v1.2.1.1 (Applied Biosystems, MDS Sciex, Toronto, Ontario, Canada). Data from LipidView were exported to Excel, group labels were added and data were imported into Markerview with lipid ID and quantification included. Data were scaled using Pareto scaling and no weighting was applied. PCA was performed in an unsupervised mode. Following PCA analysis, the top two principal components were chosen to apply principal component variable grouping [68] . Common peaks were selected with an angle delta of 40° and a minimum distance from the origin of 0.02. A minimum limit of 0.05 was applied to start a new group. Groups were assigned automatically, and the top four groups (of five) are shown on the loading plot. cAMP and cGMP quantification Synchronous trophozoite-infected RBCs were enriched using magnetic cell sorting (CS and D columns; MACS Cell Separation, Miltenyi Biotec) and counted on a haemocytometer. The cAMP levels were measured using cAMP-Screen Direct System kit (Invitrogen, Life Technologies) following the manufacturer’s instructions, while the cGMP levels were quantitated using a Biotrak cGMP competitive enzyme immunoassay kit (GE Healthcare) according to the manufacturer’s instructions (acetylation protocol). All experiments were performed in three independent replicates. Statistical analysis The data were analysed and graphed using GraphPad Prism 5.0. For gametocyte number, lipid level, cAMP and cGMP level, the data were compared using unpaired Student’s t -test. Accession codes : The mass spectrometry raw data of the lipidomics experiments have been deposited in the MetaboLights database with accession code MTBLS98 ( http://www.ebi.ac.uk/metabolights ). How to cite this article : Tran, P. N. et al. A female gametocyte-specific ABC transporter plays a role in lipid metabolism in the malaria parasite. Nat. Commun. 5:4773 doi: 10.1038/ncomms5773 (2014).